Basophils are required for the induction of Th2 immunity to haptens and peptide antigens The relative contributions of basophils and dendritic cells in Th2 skewing to foreign antigen exposure remain unclear. Here we report the ability of basophils to induce Th2 polarization upon epicutaneous sensitization with different antigens using basophil conditionally depleted Bas TRECK transgenic mice. Basophils are responsible for Th2 skewing to haptens and peptide antigens, but not protein antigens in vivo . Consistent with this, basophils cannot take up or process ovalbumin protein in significant quantities, but present ovalbumin peptide to T cells for Th2 differentiation via major histocompatibility complex class II. Intriguingly, basophils promote Th2 skewing upon ovalbumin protein exposure in the presence of dendritic cells. Taken together, our results suggest that basophils alone are able to induce Th2 skewing with haptens and peptide antigens but require dendritic cells for the induction of Th2 for protein antigens upon epicutaneous immunization. The induction of adaptive cellular immunity in the skin is initiated by antigen-presenting cells (APCs) such as dendritic cells (DCs), which provide signals through the peptide-major histocompatibility complex (MHC), costimulatory molecules, and instructive cytokines to naive T cells upon antigen encounter [1] , [2] , [3] . Distinct subsets of CD4 + T helper (Th) cells are then generated to control different types of protective immunity [4] . Th2 cells are crucial for the clearance of parasites, such as helminths, via expansion and activation of innate effector cells, including eosinophils and basophils [5] . The induction of Th2 immune responses was previously considered to depend mainly on DCs [6] . However, this dogma has recently been challenged as basophils might also have a pivotal role in this process [7] , [8] , [9] , [10] . It has been demonstrated that CD49b + FcεRI + c-Kit − basophils migrate into the draining lymph nodes (LNs) from the site of helminth infection or papain injection and act as APCs by taking up and processing antigens [7] , [9] , [10] . In addition, basophils express MHC class II and costimulatory molecules and secrete interleukin (IL)-4 and thymic stromal lymphopoietin (TSLP), which are critical for Th2 development. Thus, basophils alone are considered to induce Th2 polarization from naive T cells without requiring DCs in certain conditions. On the contrary, another group has found that IL-4-producing basophils were recruited to the mediastinal LNs upon first house dust mite exposure and contributed to the strength of the Th2 response in the lung, but that basophils could not present antigens or express the chaperones involved in antigen presentation [11] . These authors, therefore, proposed that DCs are necessary and sufficient for the induction of Th2 immunity to house dust mites in the lung without the requirement of basophils. Consistent with this, it has been reported that Th2 responses were severely impaired either after Schistosoma mansoni egg injection or during active S. mansoni infection by depletion of CD11c + cells, but not by depletion of basophils using anti-FcεRIα antibody [12] . Therefore, it is of great importance to determine whether or not, and under which conditions, basophils induce Th2 skewing to foreign antigen exposure. Recently, we demonstrated that basophils use a specific 4 kb enhancer fragment containing the 3′-untranslated region and HS4 elements to regulate Il4 gene expression [13] . Utilizing this system, we have generated mice that express human diphtheria toxin receptor under the control of HS4, which are named basophil-specific enhancer-mediated toxin receptor-mediated conditional cell knock-out (Bas TRECK) transgenic (Tg) mice [14] , [15] , [16] . In Bas TRECK Tg mice, basophils are specifically and conditionally depleted by diphtheria toxin (DT) treatment. Using these mice, we examined whether basophils induce Th2 polarization upon stimulation by different antigens such as haptens, peptides and protein antigens. We herein demonstrate that basophils are necessary for the induction of cutaneous Th2 immunity against haptens and peptide antigens but are dispensable for protein antigens. Impaired induction of IgG1 to peptide antigens We first confirmed that basophils in the bone marrow (BM) were completely depleted without affecting T cell, mast cell or DC population in Bas TRECK Tg mice after an intraperitoneal injection of DT ( Fig. 1a , and see Supplementary Figs S1A–D,S2 ). To test whether basophils are involved in the induction of cutaneous Th2 responses against protein antigens, we pretreated wild-type C57BL/6 (B6) and Bas TRECK Tg mice with DT and immunized them with ovalbumin (OVA) protein via a cutaneous patch to induce a Th2-type cutaneous immune response [17] , [18] . 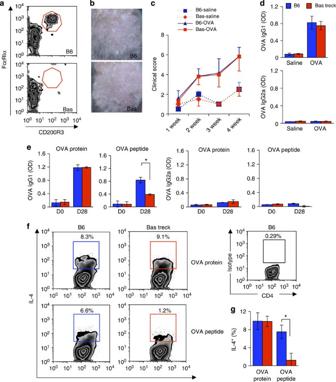Figure 1: Impaired induction of IgG1 to peptide antigens in the absence of basophils. (a) Basophils in BM in B6 and Bas TRECK mice after an intraperitoneal injection of diphtheria toxin. (b,c) Clinical manifestations (b) and clinical scores (c) of Th2-type cutaneous immune response model in DT-treated B6 and DT-treated Bas TRECK mice (n=10 per group). (d) Serum OVA-specific IgG1 levels and IgG2a in DT-treated Bas TRECK mice and DT-treated B6. (e) OVA-specific IgG1 and IgG2a responses in DT-treated B6 mice and DT-treated Bas TRECK mice in the model of immunization with OVA protein or peptide (amino acids 323–339) on day 0 and 28 mixed with alum, a strong promoter of Th2 responses. (f,g) Intracellular cytokine staining for IL-4 (f) and the frequency of IL-4+cells (g) in CD4+T cells. All data are presented as the mean±s.d. and are representative of three experiments. *P<0.05, Wilcoxon signed-rank test versus corresponding groups. Figure 1: Impaired induction of IgG1 to peptide antigens in the absence of basophils. ( a ) Basophils in BM in B6 and Bas TRECK mice after an intraperitoneal injection of diphtheria toxin. ( b , c ) Clinical manifestations ( b ) and clinical scores ( c ) of Th2-type cutaneous immune response model in DT-treated B6 and DT-treated Bas TRECK mice ( n =10 per group). ( d ) Serum OVA-specific IgG1 levels and IgG2a in DT-treated Bas TRECK mice and DT-treated B6. ( e ) OVA-specific IgG1 and IgG2a responses in DT-treated B6 mice and DT-treated Bas TRECK mice in the model of immunization with OVA protein or peptide (amino acids 323–339) on day 0 and 28 mixed with alum, a strong promoter of Th2 responses. ( f , g ) Intracellular cytokine staining for IL-4 ( f ) and the frequency of IL-4 + cells ( g ) in CD4 + T cells. All data are presented as the mean±s.d. and are representative of three experiments. * P <0.05, Wilcoxon signed-rank test versus corresponding groups. Full size image In this model, DT-treated Bas TRECK Tg (basophil-depleted) mice exhibited similar clinical manifestations to B6 mice ( Fig. 1b ). Basophils were accumulated in the skin lesion of B6 mice but absent in that of basophil-depleted mice (see Supplementary Fig. S2 ). In addition, the levels of serum OVA-specific IgG1 in basophil-depleted mice were comparable to those in B6 mice ( Fig. 1d ), whereas the production of Th1-dependent serum IgG2a was not induced by cutaneous application of OVA proteins ( Fig. 1d , right panel). To evaluate the T-cell stimulatory capacity of basophils upon protein antigen exposure, the skin draining LN cells from B6 and basophil-depleted mice after cutaneous OVA protein application were challenged with OVA protein in vitro . The incorporation of 3 H-thymidine in the presence of OVA protein was comparable between basophil-depleted mice and B6 mice (see Supplementary Fig. S3 ). The above results suggest that basophils were not essential to Th2-type immune responses induced by cutaneous application of protein antigens. Previous studies have reported that basophils, but not DCs, functioned as APC for peptide antigen-induced Th2 in vitro [9] . As such, we next compared the in vivo Th2-induction capacity of basophils upon intraperitoneal exposure to OVA protein or peptide (amino acids 323–339) mixed with alum as a strong adjuvant of Th2 responses. In this model, a significantly decreased OVA-specific IgG1 level was observed in basophil-depleted mice with OVA peptide immunization, but not with OVA protein immunization ( Fig. 1e ). At the same time point, antigen-specific IgE was undetectable in both groups due to the genetic background of these mice as B6 (refs 19 , 20 ); therefore, OVA-specific IgG1 has been used as a marker of Th2-dependent immunoglobulin in this model [19] . In addition, we examined that IgG1 production by anti-CD40 is enhanced by IL-4 ( Supplementary Fig. S4 ), which also supports the rationale that IgG1 can be used as a marker of Th2 induction. We also found that the frequency of IL-4 + cells in spleen CD4 + T cells from basophil-depleted mice was significantly lower than that from B6 mice upon OVA peptide intraperitoneal immunization, but not upon OVA protein immunization ( Fig. 1f ). The frequency of IL-4 + cells in non-T cells was also comparable between these two groups ( Supplementary Fig. S5 ). In addition, after immunized with OVA peptide, the numbers of eosinophils, CD4 + , CD4 + CD44 + CD62L + central memory, and CD4 + CD44 + CD62L − effector memory T cells in splenocytes from basophil-depleted mice were significantly decreased compared with those from B6 mice ( Supplementary Fig. S6A ). Consistently, upon immunization with OVA peptide, the messenger RNA (mRNA) levels of IL-4 and IL-13 in the mesenteric LNs in basophil-depleted mice were significantly decreased compared with those in B6 mice ( Supplementary Fig. S6B ). To further evaluate the role of basophils on T-cell differentiation after immunization with OVA protein or OVA peptide, splenocytes from B6 and basophil-depleted mice were re-challenged in the presence or absence of each antigen in vitro . Markedly decreased incorporation of 3 H-thymidine and the levels of IL-4, IL-5 and IL-13 in the culture supernatant were examined in basophil-depleted mice upon OVA peptide immunization, but not upon OVA protein immunization ( Supplementary Fig. S7A,B ). We next evaluated Th2 induction under the condition where both OVA protein and OVA peptide are used at the same time with alum. The levels of serum OVA-specific IgG1 ( Supplementary Fig. S8A–C ), the frequency of IL-4 + cells in CD4 + T from basophil-depleted mice was similar to that from B6 mice in all mol ratio (protein:peptide=2:1, 1:1, and 1:2) ( Supplementary Fig. S8D,E ). Attenuation of inflammation by repeated hapten application Haptens are one of external antigens via cutaneous penetration. A previous report demonstrated that repeated elicitation with hapten results in a shift from Th1- to Th2-mediated cutaneous inflammation, which mimics atopic dermatitis [21] . Therefore, to examine the role of basophils in hapten-induced Th2-type inflammation in the skin, we performed repeated cutaneous application of oxazolone to B6 mice and basophil-depleted mice. Although Th1-mediated delayed-type hypersensitivity as manifested by the ear swelling response to a single elicitation of oxazolone was similar between B6 and basophil-depleted mice ( Fig. 2a ), the repeated application-induced immune reaction in basophil-depleted mice was much less than that in B6 mice ( Fig. 2b ). Immediate-type hypersensitivity and late phase reaction, as manifested by the ear swelling responses 1 and 6 h after the last hapten application in basophil-depleted mice was significantly attenuated compared with those in B6 mice ( Fig. 2c ). Histological examination revealed attenuated epidermal thickening and cell infiltrations in the dermis of basophil-depleted mice ( Fig. 2d , Supplementary Table S1 ). In addition, serum oxazolone-specific IgG1 levels in basophil-depleted mice were significantly decreased compared with those in B6 mice ( Fig. 2f , left panel). Furthermore, the oxazolone-specific IgG2a levels in basophil-depleted mice were the same as those in B6 mice ( Fig. 2f , right panel). The mRNA level of TSLP in the skin lesion was increased 3 h after the last challenge in the repeated hapten application model ( Fig. 2g ). These results suggest that basophils are responsible for hapten-induced Th2 skin reaction and IgG1 induction. 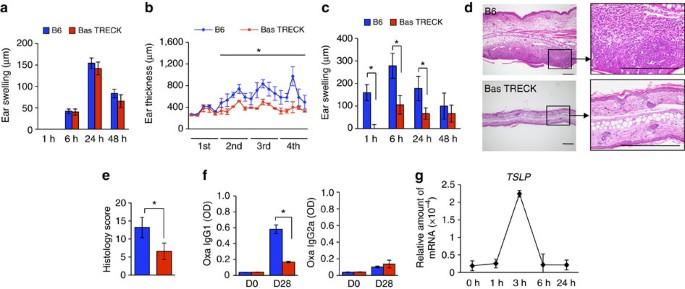Figure 2: Attenuation of ear inflammation by repeated hapten application in the DT-treated Bas TRECK mice. (a) Th1 immune response to single application of oxazolone of DT-treated B6 and DT-treated Bas TRECK (Bas -) mice. (b) Time course of repeated hapten application in these mice, (c) On fourth application, the ear swelling of these mice in the acute phase. (d) Histological examination (Scale bar, 100 μm), and scores (e). (f) Serum oxazolone-specific IgG1 and IgG2a levels in DT-treated B6 or DT-treated Bas TRECK (Bas -) mice on day 0 and 28. (g) The mRNA level ofTSLPin the skin lesion after repeated hapten application. All data are presented as the mean±s.d. (n>3) and are representative of three experiments. *P<0.05 (Wilcoxon signed-rank test) versus corresponding groups. Figure 2: Attenuation of ear inflammation by repeated hapten application in the DT-treated Bas TRECK mice. ( a ) Th1 immune response to single application of oxazolone of DT-treated B6 and DT-treated Bas TRECK (Bas -) mice. ( b ) Time course of repeated hapten application in these mice, ( c ) On fourth application, the ear swelling of these mice in the acute phase. ( d ) Histological examination (Scale bar, 100 μm), and scores ( e ). ( f ) Serum oxazolone-specific IgG1 and IgG2a levels in DT-treated B6 or DT-treated Bas TRECK (Bas -) mice on day 0 and 28. ( g ) The mRNA level of TSLP in the skin lesion after repeated hapten application. All data are presented as the mean±s.d. ( n >3) and are representative of three experiments. * P <0.05 (Wilcoxon signed-rank test) versus corresponding groups. Full size image Basophils express MHC class II and costimulatory molecules Next, we examined whether basophils express MHC class II, costimulatory molecules and chemokine receptors in draining LNs with repeated cutaneous hapten application. As reported previously, basophils were not detected in draining LNs in the steady states; however, after repeated hapten application, a significant number of CD49b + FcεRI + IgE + CD200R + c-Kit − basophils were detected ( Fig. 3a ). These basophils expressed MHC class II, CD40, CD80, CD86, CD62L, CXCR4, and CCR7, but not CCR4 ( Fig. 3b ), which suggest their potential to enter lymphoid tissues. 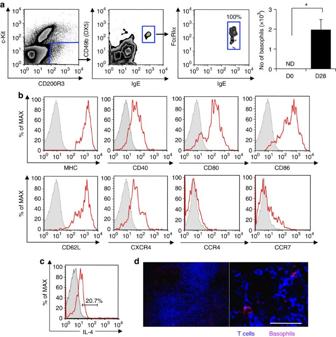Figure 3: Basophils expressed MHC class II and costimulatory molecules in the repeated hapten application model. (a) The number of CD49b+FcεRI+IgE+CD200R+c-Kit−basophils as gated (left panels), before (D0) and 28 days after repeated hapten application. (b) Expression of MHC class II, CD40, CD80, and CD86, CD62L, CCR4, CXCR4 and CCR7, on basophils (shaded histogram represents isotype-matched control antibody). (c) IL-4 production in basophils in draining LNs by means of anin vivointracellular staining assay after repeated hapten application. (d) Basophils were found in the vicinity of T cells in the T-cell zone of the draining LNs after the hapten application model. All data are presented as the mean±s.d. and are representative of three experiments. Scale bar, 50 μm. Figure 3: Basophils expressed MHC class II and costimulatory molecules in the repeated hapten application model. ( a ) The number of CD49b + FcεRI + IgE + CD200R + c-Kit − basophils as gated (left panels), before (D0) and 28 days after repeated hapten application. ( b ) Expression of MHC class II, CD40, CD80, and CD86, CD62L, CCR4, CXCR4 and CCR7, on basophils (shaded histogram represents isotype-matched control antibody). ( c ) IL-4 production in basophils in draining LNs by means of an in vivo intracellular staining assay after repeated hapten application. ( d ) Basophils were found in the vicinity of T cells in the T-cell zone of the draining LNs after the hapten application model. All data are presented as the mean±s.d. and are representative of three experiments. Scale bar, 50 μm. Full size image Basophils produce the Th2-inducing cytokine IL-4 and express TSLP after stimulation with papain in vitro and in vivo [10] . However, it remains unclear whether basophils express IL-4 in the repeated hapten application model. After repeated hapten application, a fraction of basophils produced IL-4 in draining LNs using an intracellular staining assay without any stimulation in vitro ( Fig. 3c ). As TSLP is known as a critical inducer and activator of basophils, the induction of basophils in the draining LNs ( Fig. 3a ) and their activation ( Fig. 3b ) may depend on the induction of TSLP in the draining LNs ( Fig. 2h ). In addition, basophils were found in the vicinity of T cells in the T-cell zone of the draining LNs after the hapten application model ( Fig. 3d ). Therefore, basophils accumulated in the draining LNs may be a source of IL-4 for the induction of Th2 response in the repeated hapten application model. Basophils stimulate T cells with OVA peptide Next, we examined whether basophils activate T cells in vitro . To address this issue, we used Fluo-8 for intracellular Ca 2+ staining and monitored the influx of Ca 2+ as an indicator of T-cell activation. Firstly, we confirmed that sorted basophils exhibited their characteristic multilobed nuclei by cytology ( Fig. 4a ). We incubated Fluo-8-labelled OVA-specific naive CD4 + T cells from DO11.10 T-cell antigen receptor Tg mice and CellTracker Red-labelled BM-derived basophils (BMBs) with OVA protein or OVA peptide. When an intracellular Ca 2+ level of T cells is increased, green fluorescence intensity is induced in this system. Mixing with OVA peptide induced a prominent Ca 2+ increase in T cells as shown in green fluorescence ( Fig. 4b and see Supplementary Movie 1 ). However, mixing with OVA protein did not increase intracellular Ca 2+ concentrations in T cells ( Fig. 4d ). On the other hand, DCs induced a prominent Ca 2+ increase in T cells irrespective of the presence of OVA protein or OVA peptide ( Fig. 4e ), while basophils can activate T cells only in the presence of OVA peptide ( Fig. 4d ). The capacity for inducing a calcium response in T cells in the presence of peptide is comparable between DCs and basophils ( Fig. 4d ). 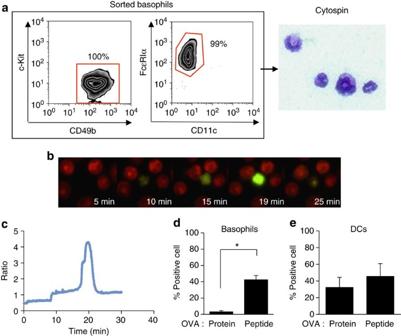Figure 4: Stimulation of T cells by BMBs with OVA peptide. (a) Sorted basophils exhibited their characteristic multilobed nuclei by cytology. (b,c) Incubation of Fluo-8-labelled naive CD4+T cells from DO11.10 and CellTracker Red-labelled BMBs with OVA protein or OVA peptide. Mixing with OVA peptide induced a prominent Ca2+increase in T cells as shown in green fluorescence (b). The fluorescence intensity was expressed as a ratio to the initial value after subtracting background fluorescence (c). (d,e) The percentage of T cells demonstrating high Ca2+concentration after mixing with OVA protein or OVA peptide in the presence of basophils (d) or DCs (e). All data are presented as the mean±s.d. and are representative of three experiments. Figure 4: Stimulation of T cells by BMBs with OVA peptide. ( a ) Sorted basophils exhibited their characteristic multilobed nuclei by cytology. ( b , c ) Incubation of Fluo-8-labelled naive CD4 + T cells from DO11.10 and CellTracker Red-labelled BMBs with OVA protein or OVA peptide. Mixing with OVA peptide induced a prominent Ca 2+ increase in T cells as shown in green fluorescence ( b ). The fluorescence intensity was expressed as a ratio to the initial value after subtracting background fluorescence ( c ). ( d , e ) The percentage of T cells demonstrating high Ca 2+ concentration after mixing with OVA protein or OVA peptide in the presence of basophils ( d ) or DCs ( e ). All data are presented as the mean±s.d. and are representative of three experiments. Full size image Basophils are unable to process protein antigens Our studies demonstrated that basophils have a role in Th2 induction with peptide antigens, but not with protein antigens. One possible reason for this is that basophils are unable to take up and process protein antigens. To explore this, we examined whether basophils take up and process OVA protein into OVA peptide. To address this issue, we used dye quenched (DQ) ovalbumin (DQ-OVA), a fluorogenic substrate for proteases, which becomes fluorescent upon hydrolysis of the DQ-OVA to single peptide by proteases. Using this system, we tested BMBs for their ability to take up and process OVA and found that CD49b + FcεRI + CD11c − BMBs could hardly take up and process OVA protein compared with bone marrow-derived dendritic cells (BMDCs) ( Fig. 5a ). 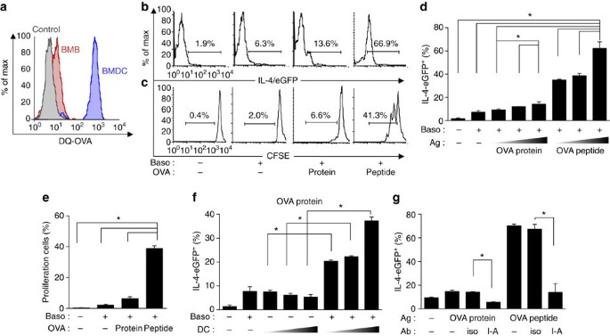Figure 5: Basophils were unable to take up and process protein antigens but induce Th2 differentiation with peptide antigensin vitro. (a) Using DQ-OVA that becomes fluorescent upon hydrolysis by phagocyte, we tested the ability to take up and process OVA by BMBs and DCs. (b–d)In vitrosystem of Th2 differentiation and T-cell stimulatory capacity. OVA-specific CD4+T cells from 4get × DO11.10 double transgenic mice (b,d) or from DO11.10 mice (c,e) were cocultured with basophils (Baso) in the presence of OVA protein or peptide. The frequency of IL-4/eGFP-positive cells, an indicator for Th2 differentiation, is shown (b,d). The populations of CFSE-diluted OVA-specific CD4+T cells after incubation for 1 day, as an indication for T-cell proliferation, were shown (c,e). (f) OVA-specific CD4+T cells were co-cultured with basophils (Baso) and/or DCs in the presence of OVA protein, and the frequency of IL-4–eGFP-positive CD4+T cells was shown. (g) The frequency of IL-4-eGFP+cells in the presence or absence of neutralizing anti-MHC class II antibody (iso: isotype-matched control, I-A: anti-MHC class II antibody). All data are presented as the mean±s.d. and are representative of three experiments. Figure 5: Basophils were unable to take up and process protein antigens but induce Th2 differentiation with peptide antigens in vitro. ( a ) Using DQ-OVA that becomes fluorescent upon hydrolysis by phagocyte, we tested the ability to take up and process OVA by BMBs and DCs. ( b – d ) In vitro system of Th2 differentiation and T-cell stimulatory capacity. OVA-specific CD4 + T cells from 4get × DO11.10 double transgenic mice ( b , d ) or from DO11.10 mice ( c , e ) were cocultured with basophils (Baso) in the presence of OVA protein or peptide. The frequency of IL-4/eGFP-positive cells, an indicator for Th2 differentiation, is shown ( b , d ). The populations of CFSE-diluted OVA-specific CD4 + T cells after incubation for 1 day, as an indication for T-cell proliferation, were shown ( c , e ). ( f ) OVA-specific CD4 + T cells were co-cultured with basophils (Baso) and/or DCs in the presence of OVA protein, and the frequency of IL-4–eGFP-positive CD4 + T cells was shown. ( g ) The frequency of IL-4-eGFP + cells in the presence or absence of neutralizing anti-MHC class II antibody (iso: isotype-matched control, I-A: anti-MHC class II antibody). All data are presented as the mean±s.d. and are representative of three experiments. Full size image Next, we used in vitro systems for Th2 differentiation and T-cell stimulatory capacity with purified OVA-specific CD4 + T cells from 4get × DO11.10 double Tg mice or from CFSE-labelled DO11.10 mice. Co-culture of BMBs and CD4 + T cells together in the presence of antigens led to IL-4-enhanced green fluorescence protein (eGFP) expression in CD4 + T cells as reported previously [8] . Although OVA peptide induced IL-4 induction in CD4 + T cells in a dose-dependent manner, OVA protein did not ( Fig. 5b ). We also performed intracellular cytokine staining for IL-4 to measure IL-4 production at the protein level. Although OVA peptide induced IL-4 production in CD4 + T cells, OVA protein did not ( Supplementary Fig. S9A,B ). Moreover, induction of Th2 responses by basophils was IL-4 dependent using neutralizing anti-IL-4 antibody ( Supplementary Fig. S9C ). T-cell stimulatory capacity was measured by a CFSE-diluted assay after incubation for 1 ( Fig. 5c ) or 3 days ( Supplementary Fig. S10 ). T-cell proliferation was enhanced by basophils in the presence of OVA peptide but not in the presence of OVA protein ( Fig. 5c , and Supplementary Fig. S10 ). As basophils cannot take up or process protein antigens ( Fig. 5a ), other cells are required to prepare peptide to be presentable. One of the candidates is DCs as it has been reported that the Th2 response to cysteine proteases requires the cooperation of DCs and basophils via reactive oxygen species-mediated signalling [22] . Therefore, we examined whether DCs support basophil-dependent Th2 induction upon exposure to protein antigens. To assess this issue, we evaluated Th2 differentiation by culturing BMBs with OVA protein in the presence or absence of BMDCs. Basophils significantly increased the frequency of IL-4–eGFP-positive CD4 + T cells upon OVA protein exposure in the presence of DCs ( Fig. 5f ). In addition, we demonstrated that the addition of a blocking antibody to MHC class II abrogated the basophil-induced Th2 responses, which rules out the possibility that the antigen has a direct effect on the T cells ( Fig. 5g ). It has recently been shown that basophils are a heterogeneous population that can be driven by either IL-3 or TSLP [15] . The number of BMBs driven by IL-3 after a repeated hapten application model was high and that after OVA cutaneous patch was rather low when compared with control mice ( Fig. 6b , left panel). Intriguingly, the numbers of BMBs driven by TSLP after both repeated hapten application and OVA cutaneous patch models were high when compared with control mice ( Fig. 6b , right panel). These results suggest that delivery of haptens promotes both IL-3 and TSLP responses, while delivery of proteins preferentially promotes TSLP responses and impairs IL-3 response. 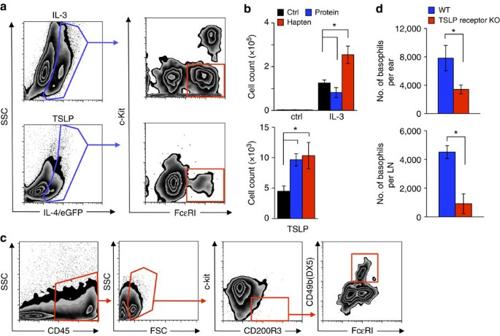Figure 6: Basophil development depends on the type of antigens. (a) BM cells were taken from 4get mice and cultured in the presence of IL-3 or TSLP. In IL-4/eGFP subsets, the FcεRI+c-Kit−basophil population is induced. (b) BM cells of mice with non-treatment, repeated hapten application (hapten) or OVA cutaneous patch (protein) were cultured in the absence (ctrl) or presence of IL-3 or TSLP, and basophil numbers were determined. (c) Basophils in the skin were detected as CD45+CD49b+FcεRI+CD200R+c-Kit−by flow cytometry. (d) The numbers of basophils in the skin and draining LNs of wild-type and TSLP receptor-deficient (KO) mice after repeated hapten application. All data are presented as the mean±s.d. and are representative of two or three independent experiments. Figure 6: Basophil development depends on the type of antigens. ( a ) BM cells were taken from 4get mice and cultured in the presence of IL-3 or TSLP. In IL-4/eGFP subsets, the FcεRI + c-Kit − basophil population is induced. ( b ) BM cells of mice with non-treatment, repeated hapten application (hapten) or OVA cutaneous patch (protein) were cultured in the absence (ctrl) or presence of IL-3 or TSLP, and basophil numbers were determined. ( c ) Basophils in the skin were detected as CD45 + CD49b + FcεRI + CD200R + c-Kit − by flow cytometry. ( d ) The numbers of basophils in the skin and draining LNs of wild-type and TSLP receptor-deficient (KO) mice after repeated hapten application. All data are presented as the mean±s.d. and are representative of two or three independent experiments. Full size image We next evaluated the nature of basophil populations using a repeated hapten application model in wild-type and TSLP receptor-deficient mice. The numbers of basophils in the skin and draining LNs in TSLP receptor-deficient mice was significantly decreased compared with those in wild-type mice ( Fig. 6c ). These results suggest that the nature of the basophil populations recruited to the skin and the draining LNs to be determined as TSLP-dependent at least in part in this model. In this study, we have demonstrated that basophils are responsible for Th2 skewing to haptens and peptide antigens but not protein antigens in vivo . We also found that basophils expressed MHC class II, CD40, CD80, CD86 and IL-4 in the hapten-induced Th2 model, but that basophils cannot take up or process OVA protein sufficiently using the DQ-OVA system. Basophils directly stimulated T cells via MHC class II/peptide complex and promoted IL-4 production in CD4 + T cells upon exposure to peptide antigens but not to protein antigens in vitro . Intriguingly, basophils sufficiently promoted Th2 skewing upon OVA protein exposure in the presence of DCs. These results suggest that basophils alone are able to induce Th2 skewing with haptens and peptide antigens but require DCs for the induction of Th2 for protein antigens. Despite recent reports that basophils act as APCs for helminth antigens or skin-injected papain [7] , [9] , [10] , another group reported that basophils do not function as APCs for inhaled house dust mite allergens [11] . Therefore, there remained a discrepancy in the ability of basophils to act as APCs. Although the experimental models differ (for example, routes of antigen administrations), we assume that this discrepancy stems from the different type of antigens, such as protein, peptide and hapten. Hapten antigens may bind to MHC class II on the surface of basophils directly, and peptide can be acquired and presented by basophils, while protein antigens are not presented efficiently by basophils because they are hardly digested by these cells. In fact, previous reports demonstrated that basophils promote Th2 induction using OVA peptide but not OVA protein in vitro [7] , [9] . The protease allergen papain reaches the LNs after its cutaneous immunization and induces MHC class II expression on basophils in accord with preparing OVA peptide antigens from OVA protein in vivo [9] . Another group has reported that basophils pulsed with anti-2, 4-dinitrophenyl (DNP IgE) enhance Th2 skewing upon exposure to DNP-conjugated OVA by taking up DNP-OVA–IgE anti-DNP immune complexes [7] . Although house dust mites also contain cysteine protease activity, they are not sufficient for Th2 induction as they do not upregulate MHC class II on basophils in this model, even though cysteine proteases may function to generate peptide antigens from protein antigens in vivo [11] . Herein, we have shown that DCs support basophils to increase the frequency of IL-4–eGFP-positive CD4 + T cells. As basophils cannot take up or process protein antigens efficiently, DCs may prepare peptide to be presented by basophils or may promote basophils to produce IL-4 to skew Th2. In line with this, our recent study has demonstrated that Langerhans cells, an epidermal DC subset, mediate epicutaneous sensitization with OVA protein antigens to induce Th2-type immune responses [23] . In addition, Th2 reactions are reduced upon sensitization with protein antigens or Schistosome infections using a CD11c-depletion model [11] , [12] ; therefore, DCs seem to be necessary for Th2 induction both in vivo and in vitro upon protein antigen exposure. As basophils were found in the vicinity of T cells in the T-cell zone of the draining LNs, basophils, T cells and DCs may act towards Th2 induction in a coordinated way. In future, it will be intriguing to further evaluate whether DCs present peptide to basophils directly or by trogocytosis. Taken together, basophils seem to be important for Th2 induction when stimulated with OVA peptide or hapten alone. Consistently, basophils hardly take up and process protein antigen compared with DCs ( Fig. 5a ). In line with this, DCs seem to be sufficient for Th2 induction when stimulated with OVA protein or both OVA protein and OVA peptide in vivo . Intriguingly, however, our in vitro data suggest that basophils support induction of Th2 responses upon OVA protein exposure in the presence of DCs ( Fig. 5f ). Therefore, DCs can to be sufficient for Th2 induction in the context of complex inflammatory environments like post- S. mansoni infection, where presumably various different ratios of small soluble antigens and larger proteins are present. A fraction of basophils have the capacity to produce IL-4 in draining LNs in our model ( Fig. 3c ). Previously, Sullivan et al . [24] demonstrated that basophils produce IL-4 only in the lung tissues but not in the draining LNs when they used an Nippostrongylus brasiliensis infection model. In this study, we used a repeated hapten application model in which mice were immunized epicutaneously. We previously demonstrated that epidermal keratinocytes express a Th2 inducer TSLP and that TSLP-TSLP signalling is essential for IgE induction [23] . In addition, the number of basophils in the draining LNs in TSLP receptor-deficient mice was decreased compared with that in wild-type mice ( Fig. 6d ). At present, we still do not know how IL-4 is produced by basophils in the draining LNs in our model, but we assume that the TSLP-dependent basophils might be involved in our context. Our results suggest that delivery of haptens and proteins differentially regulate TSLP and IL-3 response of basophils ( Fig. 6b ), which would provide critical insight into the reasons why some infections (which may be IL-3 or TSLP inducing) may be more DC- or basophil- dependent. It has been reported that serum IgE levels are one of the major factors that influence basophil populations [25] . Antigen-specific IgE was not detected in OVA protein or peptide sensitization models. On the other hand, TSLP is known to be elevated in the skin lesions of atopic dermatitis, upon barrier disruption, or by protease-containing antigen-exposure [26] , [27] , [28] . These conditions may affect heterogeneity in the basophil lineage (TSLP/IL-3), which has a role in each of these systems. It will be interesting to investigate the amounts of IL-3 and TSLP in situ upon stimulation with a variety of foreign antigens, including hapten, protein and bacteria, in a context-dependent manner. Mice Mice expressing human diphtheria toxin receptor under the control of 3′-UTR element in the Il4 locus were generated for Bas TRECK by a transgenic strategy as reported previously [14] , [16] . C57BL/6 (B6) and BALB/c mice were purchased from Japan SLC (Shizuoka, Japan). We treated C57BL/6 (B6) mice with DT as control and Bas TRECK Tg mice with DT as basophil-depleted mice. DO11.10 transgenic mice and 4get mice were purchased from Jackson Laboratory (Bar Harbor, ME). TSLP receptor-deficient mice (BALB/c) were kindly provided by Dr Steven Ziegler (University of Washington). For DT treatment, mice were injected intraperitoneally with 500 ng of DT per mouse on the first day. Then Bas-TRECK mice were treated at 3-day intervals [16] . Eight- to ten-week-old female mice were used for all of the experiments and were bred in specific pathogen-free facilities at Kyoto University. All experimental procedures were approved by the institutional animal care and use committee of the Kyoto University Graduate School of Medicine. Reagents and antibodies We purchased oxazolone from Wako Pure Chemical Industries, Ltd. (Osaka, Japan), OVA from Sigma-Aldrich (St Louis, MO), OVA peptide from MBL (Nagoya, Japan), and DQ-OVA from Invitrogen (Carlsbad, CA). FITC-, PE-, PE-Cy7-, APC-, APC-7- and Pacific Blue-conjugated 145-2C11 (anti-CD3), N418 (anti-CD11c), 1C10 (anti-CD40), DX5 (anti-CD49b), 16-10A1 (anti-CD80), GL1 (anti-CD86), 2B8 (anti-CD117), M5/114.15.2 (anti-MHC class II), MEL-14 (anti-CD62L), eBioL31 (anti-CD207), 2B11 (anti-CXCR4), 4B12 (anti-CCR7), IgE (23G3), blocking antibody to IL-4 (11B11) (eBioscience, San Diego, CA), Ba103 (anti-CD200R3) (Hycult Biotech, Plymouth Meeting, PA), IL-4 (BVD4-1D11) (BD, Franklin Lakes, NJ), TUG8 (anti-MCP8) and 2G12 (anti-CCR4) (BioLegend, San Diego, CA) were purchased. Intracellular staining was performed with Cytofix/Cytoperm reagents (BD) according to the manufacturer’s instructions and analysed with FACS Fortessa (BD). For the pretreatment of IL-4 staining in CD4 + T cells, splenocytes were collected and incubated with PMA (20 ng ml −1 ) and ionomycin (1 μM) for four hours. For the in vivo intracellular staining assay [29] , mice were pretreated with intravenous injection with 500 μl of PBS solution containing 100 μg monensin (Sigma-Aldrich) for 6 h. Epicutaneous sensitization and clinical severity Epicutaneous sensitization with protein antigens, the clinical severity scoring of skin lesions, and the histological scoring were performed as reported previously [23] , [30] . In brief, mice were anesthetized with diethylether (Nacalai Tesque, Kyoto, Japan) and shaved with an electric shaver (THRIVE Co. Ltd., Osaka, Japan). A single skin site on each mouse was tape-stripped five times with adhesive cellophane tape (Nichiban, Tokyo, Japan). One-hundred milligram of OVA in 100 μl of normal saline was placed on the patch-test tape (Torii Pharmaceutical Co., Ltd., Tokyo, Japan). Each mouse had a total of three 2-day exposures to the patch, separated by 1-day intervals. The total clinical score for skin lesions was designated as the sum of individual scores (graded none as 0, mild as 1, moderate as 2 and severe as 3) for the symptoms of pruritus, erythema, oedema, erosion and scaling. Immunohistochemical analysis was performed as reported previously [14] . Th2 induction model and ELISA B6 and basophil-depleted mice were sensitized with intraperitoneal injections of alum (20 mg ml −1 ) with OVA protein (100 μg ml −1 ) or OVA peptide (10 μg ml −1 ) on day 0, day 14, day 21 and day 28. Total serum IgE/IgG1/IgG2a levels were measured using a Bio-Rad (Hercules, CA) Luminex kit according to the manufacturer’s instructions. To measure OVA/oxazolone-specific IgE/IgG1/IgG2a levels, the appropriate mouse IgE/IgG1/IgG2a ELISA kit (Bethyl Laboratories, Montgomery, TX) was used with slight modifications. Absorbance was measured at 450 nm. The difference between the sample absorbance and the mean of negative control absorbance was taken as the result. Repeated oxazolone application Repeated oxazolone treatment was performed essentially as described [31] . Mice treated with vehicle without oxazolone were used as control. Ear thickness was measured using a micrometre before, 1, 6, 24 and 48 h after challenge to assess inflammation. Ears were then collected for histology. Quantitative PCR analysis Quantitative PCR analysis was performed as reported previously [30] . The primer sequences for TSLP : 5′-ACGGATGGG GCTAACTTACAA-3′ (forward) and 5′-AGTCCTCGATTTGCTCGAACT-3′ (reverse). Generation of BMDC and BMB Complete RPMI (cRPMI), RPMI 1640 medium (Sigma, St Louis, MO) containing 10% fetal calf serum (FCS) (Invitrogen), was used as the culture medium. For BMDC induction, 5 × 10 6 BM cells from BALB/c mice were cultured supplemented with 10 ng ml −1 recombinant murine GM-CSF (PeproTech, Rocky Hill, NJ) for 5 days (>90% expressed CD11c). For BMB induction by IL-3, 5 × 10 6 BM cells from BALB/c mice were cultured supplemented with 10 ng ml −1 recombinant murine IL-3 (PeproTech) containing 20% FCS for 10 days. In some experiments, for BMB induction by TSLP or IL-3, BM cells from 4get mice were cultured in the presence of 1 μg ml −1 of TSLP for 5 days as reported previously [15] . Cytoplasmic Ca 2+ imaging T cells were incubated with 5 μM Quest Fluo-8 AM (ABD Bioquest, CA), and BMBs and BMDCs were stained with 2 μM CellTracker Red (Invitrogen). The Fluo-8 image and the transmission image were recorded every 10 s using a back-thinned electron multiplier charge-coupled device (CCD) camera (ImagEM, Hamamatsu Photonics, Japan) and a microscope (Eclipse Ti, Nikon, Japan). The fluorescence intensity was expressed as a ratio to the initial value after subtracting background fluorescence. Processing of OVA and Th2 differentiation For measuring internalization and processing of OVA, 1 × 10 6 cells of BMDCs or BMBs were incubated with DQ-OVA (5 μg ml −1 , Invitrogen) for 1 h and analysed with FACS Fortessa. For Th2 differentiation in vitro , naive CD4 + T cells were sorted by microbeads (Miltenyi Biotec, Bergisch Gladbach, Germany) and were plated at a density of 5 × 10 5 cells per ml in the presence of various ratios of OVA protein (2, 10, 50 μg ml −1 ), OVA peptide (0.4, 2, 10 μg ml −1 ) and/or BMDCs (1 × 10 4 , 2 × 10 4 , 1 × 10 5 cells) in RPMI medium with 10% FCS for 3 days, standard supplements and IL-3 (30 ng ml −1 ) for basophil survival. BMBs were sorted with anti-PE-ckit and anti-PE-CD11c by anti-PE microbeads and plated at a ratio of 1:5 with CD4 + T cells. Statistical analysis Unless otherwise indicated, data are presented as the means±s.d. and are representative of three independent experiments. P -values were calculated with the Wilcoxon signed-rank test. P -values <0.05 are considered to be significantly different between basophil-depleted mice and corresponding B6 mice and are marked by an asterisk in the figures. How to cite this article: Otsuka, A. et al . Basophils are required for the induction of Th2 immunity to haptens and peptide antigens. Nat. Commun. 4:1739 doi: 10.1038/ncomms2740 (2013).